Artemisinin-resistantPlasmodium falciparumclinical isolates can infect diverse mosquito vectors of Southeast Asia and Africa Artemisinin-resistant Plasmodium falciparum parasites are rapidly spreading in Southeast Asia, yet nothing is known about their transmission. This knowledge gap and the possibility that these parasites will spread to Africa endanger global efforts to eliminate malaria. Here we produce gametocytes from parasite clinical isolates that displayed artemisinin resistance in patients and in vitro , and use them to infect native and non-native mosquito vectors. We show that contemporary artemisinin-resistant isolates from Cambodia develop and produce sporozoites in two Southeast Asian vectors, Anopheles dirus and Anopheles minimus , and the major African vector, Anopheles coluzzii (formerly Anopheles gambiae M). The ability of artemisinin-resistant parasites to infect such highly diverse Anopheles species, combined with their higher gametocyte prevalence in patients, may explain the rapid expansion of these parasites in Cambodia and neighbouring countries, and further compromise efforts to prevent their global spread. Artemisinin (ART) resistance in P. falciparum threatens to decrease the efficacy of all ART combination therapies (ACTs) [1] , [2] , severely compromising global efforts to eliminate this malaria parasite. Indeed, ART resistance has quickly led to the failure of dihydroartemisinin-piperaquine, the current frontline ACT for falciparum malaria in Western Cambodia [3] , [4] . Although ART-resistant P. falciparum parasites have emerged and rapidly expanded in Cambodia and other Greater Mekong Subregion (GMS) countries [5] , [6] , [7] , [8] , [9] , [10] , and may spread to Africa, nothing is known about their transmission to native or non-native mosquito vectors. Two recent findings in Western Cambodia, however, have important implications for the transmission of these parasites. First, patients with ART-resistant parasites more often present with gametocytemia, or develop gametocytemia while taking an ACT, than those with ART-sensitive parasites [9] , suggesting that ART-resistant parasites have increased transmission potential. Second, population genetics studies of P. falciparum clinical isolates have revealed that ART-resistant parasites often undergo population expansions, resulting in highly structured founder populations that are as differentiated from each other as they are from African parasites [11] , [12] . These founder populations display slow parasite clearance following ACTs in patients [11] , [12] , show resistance to ART in the Ring-stage Survival Assay in vitro [13] , [14] and carry different kelch13 ( K13 ) mutations [8] , [12] that confer ART resistance [15] , [16] . The GMS hosts a great diversity of anopheline vectors capable of transmitting malaria [17] , [18] , [19] . The roles of these vectors in transmitting parasites from several ART-resistant founder populations and the ART-sensitive core population of Cambodia have not been investigated. Given that parasite clones within each ART-resistant founder population are nearly genetically identical [11] , [12] and that P. falciparum strains can vary remarkably in their infectivity to Anopheles species in vitro [20] , [21] , [22] , we hypothesized that adaptation to native Anopheles species influences the spread of ART-resistant founder populations within the GMS and that failure to infect non-native vectors prevents their transmission in other regions. Characterizing the ability of ART-resistant parasites to infect vectors in Africa is particularly critical in assessing the risks of their spread to this continent, where most of the world’s malaria transmission, morbidity and mortality occur. The anopheline fauna in Cambodia and other GMS countries includes a large number of vector species, entirely distinct from the relatively few vector species in malaria-hyperendemic settings of Africa. The diversity of Anopheles species in the GMS and the lack of knowledge about their bionomic characteristics complicate efforts to delimit, restrict and disrupt malaria transmission patterns in this region. Moreover, the predominantly outdoor-biting and outdoor-resting behaviors of these mosquitoes undermine vector control strategies that rely on indoor interventions, such as insecticide-treated bednet use and indoor residual spraying [17] , placing the burden of malaria control primarily on clinical interventions that have repeatedly failed owing to drug resistance [19] . Although An. dirus is believed to be the primary malaria vector in Cambodia, and other species including An. minimus , An. maculatus and An. barbirostris are considered secondary vectors, the current roles of these vectors in transmitting malaria have not been adequately defined. To investigate the current transmission dynamics of P. falciparum , we produced gametocytes from parasite clinical isolates that displayed ART resistance or sensitivity in patients [6] , [11] , [12] and in vitro [13] , [14] , and used them to infect native and non-native mosquito vectors. Here we show that contemporary ART-resistant isolates from Cambodia develop and produce sporozoites in two Southeast Asian vectors, An. dirus and An. minimus , and the major African vector, An. coluzzii (formerly An. gambiae M). The ability of ART-resistant parasites to infect such diverse anophelines, combined with their higher gametocyte prevalence in patients [9] , may be contributing to the rapid expansion of these parasites in Cambodia and other GMS countries. These findings pose serious challenges to eliminating ART-resistant malaria from Southeast Asia and preventing its spread to Africa. Despite the alarming potential of ART resistance spreading throughout the GMS and to Africa, we still do not know whether Cambodian founder populations can infect major Southeast Asian malaria vectors or An. coluzzii and An. gambiae [23] , the two major African vectors. To address these knowledge gaps, we used a standard membrane feeding assay to assess whether nine Cambodian P. falciparum clinical isolates can infect five different Anopheles species. P. falciparum mosquito-infective gametocytes were induced and matured in culture for 2 weeks and fed to mosquitoes using glass feeders with an artificial membrane. Fed mosquitoes were dissected 1 week later to evaluate oocyst infection of their midguts (a standard measurement of mosquito infection), and the salivary glands of a subset of these mosquitoes were examined an additional 1 week later for the presence of human-infective sporozoites. Parasite isolates were tested in recently adapted colonies of An. dirus from Pursat Province, Western Cambodia, and An. coluzzii from Theirola, Mali; a long-term-adapted colony of An. minimus from Western Thailand; and two long-term-adapted Anopheles stephensi Nijmegen and An. gambiae G3 lines. These latter two lines are commonly used in laboratory investigations because they are highly permissive to infection by multiple P. falciparum strains, a phenotype for which they were artificially selected decades ago. These five vector species are highly evolutionarily distinct, having diverged from each other more than 30 million years ago [24] . For mosquito infection experiments, we selected three parasites from the ART-sensitive core population (KH-C) in Ratanakiri Province, Eastern Cambodia, which carry the wild-type (WT) K13 allele, and six parasites from three ART-resistant founder populations in Pursat, which carry different mutant K13 alleles: WKH-F02/R539T ( n =3), WKH-F04/Y493H ( n =2) and WKH-F03/C580Y ( n =1) [11] , [12] . 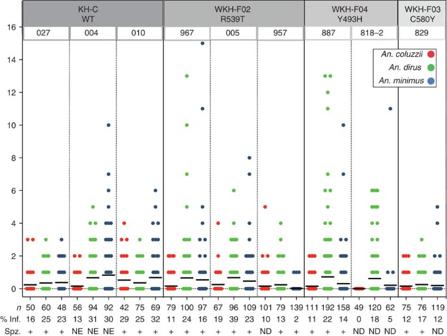Figure 1: Infection of differentAnophelesspecies by CambodianP. falciparumclinical isolates. Three ART-sensitive parasites carrying WTK13alleles (KH-C/WT) and six ART-resistant parasites from three Western Cambodian founder populations carrying different mutantK13alleles (WKH-F02/R539T, WKH-F04/Y493H and WKH-F03/C580Y) were used to infect malaria vectors of Africa (An. coluzzii) and Southeast Asia (An. dirusandAn. minimus) in parallel. Infection intensity was measured by counting the number of parasite oocysts per mosquito midgut in individual mosquitoes 8 days after they were fed gametocyte-infected erythrocytes. Each dot represents the oocyst count in a single mosquito midgut; black bars indicate the mean number of oocysts per midgut for all mosquitoes dissected. At least four independent feeds were performed for each parasite–mosquito combination.n, number of fed mosquitoes checked for oocysts; % Inf., proportion of fed mosquitoes with ≥1 oocyst; Spz., sporozoites were found in the salivary glands of a subset of mosquitoes dissected on day 14 after feeding (+), or their presence could not be determined (ND), typically owing to low infection rates, or were not examined (NE). Most of these isolates were previously found to be either ART sensitive or ART resistant in patients [6] , in vitro [14] or both ( Table 1 ). With a single exception, all nine parasite isolates infected all five mosquitoes tested ( Fig. 1 and Supplementary Fig. 1 ). Consistent with previous studies of laboratory-based infections of Southeast Asian and African vectors with P. falciparum clinical isolates [22] , [25] , [26] , [27] , mosquitoes infected with our Cambodian P. falciparum isolates showed relatively low oocyst counts: one or two oocysts per infected midgut were typically seen, whereas more than five oocysts per infected midgut were uncommon and infection prevalence was usually <30% ( Fig. 1 and Supplementary Figs 1 and 2 ). We found no indication that any of the five mosquito lines were refractory to infection; that is, we did not observe melanized parasites in the midguts of non-infected mosquitoes or infected mosquitoes with low numbers of oocysts. Table 1 Characteristics of Cambodian P. falciparum clinical isolates used to infect Anopheles species. Full size table Figure 1: Infection of different Anopheles species by Cambodian P. falciparum clinical isolates. Three ART-sensitive parasites carrying WT K13 alleles (KH-C/WT) and six ART-resistant parasites from three Western Cambodian founder populations carrying different mutant K13 alleles (WKH-F02/R539T, WKH-F04/Y493H and WKH-F03/C580Y) were used to infect malaria vectors of Africa ( An. coluzzii ) and Southeast Asia ( An. dirus and An. minimus ) in parallel. Infection intensity was measured by counting the number of parasite oocysts per mosquito midgut in individual mosquitoes 8 days after they were fed gametocyte-infected erythrocytes. Each dot represents the oocyst count in a single mosquito midgut; black bars indicate the mean number of oocysts per midgut for all mosquitoes dissected. At least four independent feeds were performed for each parasite–mosquito combination. n , number of fed mosquitoes checked for oocysts; % Inf., proportion of fed mosquitoes with ≥1 oocyst; Spz., sporozoites were found in the salivary glands of a subset of mosquitoes dissected on day 14 after feeding (+), or their presence could not be determined (ND), typically owing to low infection rates, or were not examined (NE). Full size image Supplementary Fig. 2 shows differential oocyst prevalence between five mosquito species infected with each of nine parasite isolates. For some isolates (004, P =0.0120; 005, P =0.0137; 957, P =0.0300; 887, P =0.0021; analysis of deviance), there were significant differences in infection prevalence between An. dirus , An. minimus and An. coluzzii ( Fig. 2 ). Only the effect for isolate 887, however, remained significant after adjusting for multiple comparisons ( P adj =0.019). For a different set of isolates (010, P =0.0327; 967, P =0.0022, P adj =0.0157; 887, P =0.0144; 818-2, P =0.0011, P adj =0.0087; 829, P <0.0001, P adj <0.0001), there were significant differences in infection prevalence between An. stephensi Nijmegen and An. gambiae G3 ( Supplementary Fig. 3 ). These differential mosquito species effects on infection prevalence do not appear to cluster by founder population and we see no significant clustering ( P =0.85 for Fig. 2 and P =0.26 for Supplementary Fig. 3 ; permutation test). These differences in infection prevalence suggest that highly related parasites within a given founder population possess genetic differences that mediate differential infection of anophelines. When considering only infected mosquitoes, we found that no isolate showed a significant difference in oocyst intensity between An. dirus , An. minimus and An. coluzzii (overall P =0.1651; analysis of variance test of interaction) or between An. stephensi Nijmegen and An. gambiae G3 (overall P =0.2411), but this lack of significance may be attributable to low infection rates. 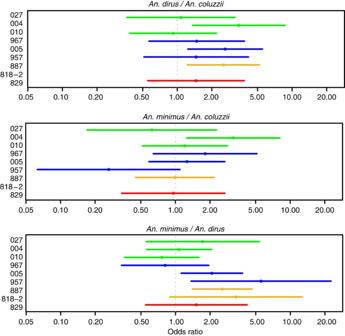Figure 2: Relative infectivity ofP. falciparumclinical isolates toAn. dirus,An. minimusandAn. coluzzii. Estimates (points) and 95% confidence intervals (lines) for odds ratios of any oocyst infection, done by a separate logistic regression for each isolate that controls for replicate feeds. The top panel shows the odds for infection ofAn. dirusover the odds forAn. coluzzii, the middle panel shows the odds forAn. minimusover the odds forAn. coluzziiand the bottom panel shows the odds forAn. minimusover the odds forAn. dirus.Isolates are colored according to population: KH-C/WT (green), WKH-F02/R539T (blue), WKH-F04/Y493H (yellow) and WKH-F03/C580Y (red). Figure 2: Relative infectivity of P. falciparum clinical isolates to An. dirus , An. minimus and An. coluzzii . Estimates (points) and 95% confidence intervals (lines) for odds ratios of any oocyst infection, done by a separate logistic regression for each isolate that controls for replicate feeds. The top panel shows the odds for infection of An. dirus over the odds for An. coluzzii , the middle panel shows the odds for An. minimus over the odds for An. coluzzii and the bottom panel shows the odds for An. minimus over the odds for An. dirus. Isolates are colored according to population: KH-C/WT (green), WKH-F02/R539T (blue), WKH-F04/Y493H (yellow) and WKH-F03/C580Y (red). Full size image Subsets of mosquitoes were also examined 2 weeks after parasite infection for the presence of salivary-gland sporozoites, the human-infective stage of P. falciparum in natural settings. We observed salivary-gland sporozoites in 153 of 216 (71%) mosquitoes, including An. dirus , An. minimus and An. coluzzii , infected with ART-resistant isolates from all three founder populations ( Fig. 1 ). In 90% of preparations, we found sporozoites to be motile—an indication of viability. Other subsets of infected mosquitoes showed no sporozoites, but this is probably explained by our observations of unruptured oocysts and inability to detect sporozoites due to low infection rates (that is, there were no infected mosquitoes in the subset checked for sporozoites). All seven isolates we examined produced sporozoites in An. stephensi Nijmegen and An. gambiae G3 ( Supplementary Fig. 1 ). Infections of An. dirus and An. coluzzii with two ART-resistant isolates (887 and 967) showed comparable numbers of salivary-gland sporozoites per infected female mosquito ( Supplementary Fig. 4 ). Collectively, our data indicate that all nine ART-resistant and ART-sensitive parasites readily infect and produce sporozoites in highly diverse Anopheles species. Although infections with multiple independently reared colonies of each Anopheles species may be necessary to determine their species-specific susceptibility to these parasite isolates, our preliminary study has two important strengths. First, all of the ART-resistant clinical isolates we studied were clonal members of founder populations, which are the most relevant sources of the parasites that initially emerged and subsequently spread in the natural setting of Western Cambodia—the epicenter of ART resistance in Southeast Asia. Second, we tested two recently colonized vectors— An. dirus from Western Cambodia and An. coluzzii from Mali—that are arguably more relevant to the current potential spread of ART-resistant parasites in Southeast Asia and Africa, respectively, than the laboratory-selected, highly permissive An. stephensi Nijmegen and An. gambiae G3 lines that are commonly used in infection studies. Our data show that several contemporary parasite isolates from Cambodia differentially infect Anopheles species in a laboratory setting. Although elucidating the molecular basis of this finding requires further investigation, we have excluded a possible role for polymorphism in the Pfs47 gene ( PF3D7_1346800 ), which was recently shown to mediate the differential infectivity of the NF54, GB4 and 7G8 P. falciparum strains in the An. stephensi Nijmegen and An. gambiae G3 lines [28] , [29] . All six ART-resistant isolates we tested possess the same Pfs47 haplotype ( Fig. 3 and Supplementary Table 1 ), the most common among 22 haplotypes identified in our recent collection of 516 Cambodian parasite isolates ( Supplementary Table 2 ). Similarly, the three ART-sensitive isolates we tested share the same Pfs47 haplotype ( Fig. 3 and Supplementary Table 1 ), the third most common in our parasite collection ( Supplementary Table 2 ). 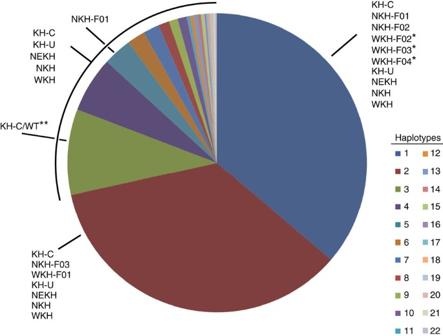Figure 3: Distribution ofPfs47haplotypes among CambodianP. falciparumclinical isolates. ThePfs47alleles of 516 parasite isolates were genotyped against the 3D7 reference genome (ver. 3). This procedure identified 22 different haplotypes, which are listed in order of decreasing prevalence in our sample collection (Supplementary Tables 1 and 2). ThePfs47haplotypes of parasites from the core population of Eastern Cambodia (KH-C) and multiple founder populations of Western (WKH), Northern (NKH) and Northeastern (NEKH) Cambodia are indicated. The six ART-resistant isolates we used in our study belong to the WKH-F02, WKH-F04 and WKH-F03 founder populations (*), all of which possess the samePfs47haplotype 1 (Supplementary Tables 1 and 2). The three ART-sensitive isolates we used belong to the KH-C/WT population (**) and have the samePfs47haplotype 3 (Supplementary Tables 1 and 2). It is noteworthy thatPfs47haplotype 1 is present in four of five ART-resistant founder populations, whereas all 22Pfs47haplotypes are present in ART-sensitive isolates (Supplementary Table 2). Figure 3: Distribution of Pfs47 haplotypes among Cambodian P. falciparum clinical isolates. The Pfs47 alleles of 516 parasite isolates were genotyped against the 3D7 reference genome (ver. 3). This procedure identified 22 different haplotypes, which are listed in order of decreasing prevalence in our sample collection ( Supplementary Tables 1 and 2 ). The Pfs47 haplotypes of parasites from the core population of Eastern Cambodia (KH-C) and multiple founder populations of Western (WKH), Northern (NKH) and Northeastern (NEKH) Cambodia are indicated. The six ART-resistant isolates we used in our study belong to the WKH-F02, WKH-F04 and WKH-F03 founder populations (*), all of which possess the same Pfs47 haplotype 1 ( Supplementary Tables 1 and 2 ). The three ART-sensitive isolates we used belong to the KH-C/WT population (**) and have the same Pfs47 haplotype 3 ( Supplementary Tables 1 and 2 ). It is noteworthy that Pfs47 haplotype 1 is present in four of five ART-resistant founder populations, whereas all 22 Pfs47 haplotypes are present in ART-sensitive isolates ( Supplementary Table 2 ). Full size image As all nine parasites infected nearly every anopheline we tested, it is possible that these two Pfs47 haplotypes do not strongly restrict parasite–mosquito compatibility in Cambodia and may not prevent the spread of similar isolates within Africa. As ART-resistant founder populations circulate in areas of high anopheline diversity, they may have been naturally selected on a genetic background of Pfs47 alleles (or other genetic determinants) that collectively confer the ability to infect most native anophelines and thus to efficiently spread. As all ART-resistant founder populations possess either of the two most common Pfs47 haplotypes we have observed in Cambodia ( Fig. 3 and Supplementary Tables 1 and 2 ), the lack of Pfs47 polymorphism among our ART-resistant isolates may simply reflect founder effects. This is because Pfs47 is in close proximity to K13 on chromosome 13 and thus is likely to be genetically linked with the K13 haplotype in founder populations. In summary, our finding that all five mosquito lines are susceptible to parasite infection suggests that native and non-native vectors are likely to be competent in transmitting ART-resistant and ART-sensitive P. falciparum populations beyond Cambodia. Detailed studies of field-relevant parasites and vectors, including whole-genome sequence analyses of multiple Southeast Asian P. falciparum isolates [11] , [12] , [30] and recently colonized Anopheles species [24] , will undoubtedly help unravel the complex genetic and behavioral determinants of malaria transmission in regions where vector species are poorly characterized. Our finding that highly differentiated ART-resistant parasites infect highly diverse Anopheles species unveils a significant unanticipated challenge to the elimination of malaria in Southeast Asia and the prevention of ART-resistant malaria in Africa. Parasite culture The P. falciparum isolates we used in this study are as follows: three parasites from the ART-sensitive core population (KH-C) in Ratanakiri that carry the WT K13 allele and six parasites from three ART-resistant founder populations in Pursat that carry different mutant K13 alleles: WKH-F02/R539T ( n =3), WKH-F04/Y493H ( n =2) and WKH-F03/C580Y ( n =1) [11] , [12] ( Table 1 ). P. falciparum clinical isolates were adapted and maintained in O + human erythrocytes (Interstate Blood Bank Inc., Memphis, TN) in RPMI 1640 medium containing HEPES, 25 mM sodium bicarbonate, 50 mg l −1 hypoxanthine and 10% heat-inactivated human serum at 1–2% parasitemia. Gametocytogenesis was induced by initiating cultures at high parasitemia and then diluting them to 3–6% parasitemia at 5% hematocrit in 20 or 30 ml of culture medium. Cultures were incubated at 37 °C in an atmosphere of 5% O 2 , 5% CO 2 and 90% N 2 , and medium was changed daily for 14–16 days. Mosquitoes The An. dirus A colony was isolated from Veal Veng District, Pursat Province, Western Cambodia, in July 2011. Unlike most An. dirus A colonies, this colony mates freely in our insectary. The identity of this colony was confirmed by sequencing the ribosomal DNA ITS2 region. Its rDNA sequence was 100% identical to a previously reported An. dirus A rDNA sequence [31] . The An. minimus A colony was obtained from the Malaria Research and Reference Reagent Resource Center as part of the BEI Resources Repository, NIAID, NIH: An. minimus MINIMUS1, MRA-729, deposited by M.Q. Benedict. This colony was isolated in Mae Sot, Western Thailand, in 1990. The An. coluzzii (formerly An. gambiae M) colony was isolated from Theirola, Mali, in November 2012. The identity of this colony was confirmed by genotyping via PCR and Hha -I digestion [32] . The An. stephensi Nijmegen colony was obtained from Joep Meuwissen, Catholic University of Nijmegen, The Netherlands, in 1985. The An. gambiae G3 colony, a laboratory line comprising a mixture of An. gambiae M and S forms, was obtained from George Davidson, London School of Hygiene and Tropical Medicine, in 1973. Mosquito feeds Mosquitoes were reared at low density (200 per 26 × 32 cm tray or 500 per 38 × 52 cm tray) at 27 °C and 75% humidity on a 12:12 light–dark cycle. Three- to 6-day-old mosquitoes, prepared at a density of 30–60 per pint container, were artificially fed using glass feeders heated to 37 °C and covered with paraffin film or hog gut membranes. Feeders were loaded with 400 μl of feed mixture diluted to ∼ 0.15% mature stage-V gametocytemia. Feed mixtures were fed to all five Anopheles colonies in parallel and each feed was done at least four times. The presence of exflagellating gametocytes in the feed mixture was confirmed before and after feeding. Mosquito dissections Parous female mosquitoes were dissected on day 8 post infection and their midguts stained with 0.2% mercurochrome in water and examined under a compound microscope. A subset of mosquitoes infected with each isolate was set aside and examined on day 14 post infection for the presence of sporozoites in salivary glands, which were dissected and ruptured under a cover slip and examined by microscopy at × 40 magnification. The number of sporozoites in the salivary glands of infected female mosquitoes was estimated using a hemocytometer. Salivary glands were dissected from females with at least one ruptured oocyst at 16–18 days post infection, placed in 40 μl of PBS and pipetted repeatedly to release sporozoites into solution. Ten microlitres of this sporozoite suspension were loaded onto a hemocytometer, sporozoites in each 4 × 4 grid were counted and standard calculations were performed to estimate the number of sporozoites per infected female mosquito. Statistical analysis Prevalence effects were modelled using logistic regression that controlled for replicate feed effects. Replicates that added no information about differential mosquito species infection rates (for example, replicates where no oocysts were observed in any mosquito species) were removed from that analysis. Inference used Wald’s confidence intervals for individual odds ratio effects and analysis of deviance for P -values of overall effect. The notation P adj refers to Holm’s adjusted P -values used to adjust for the fact that nine isolates were tested [33] . To test for the clustering founder effect, we used a permutation test, where the test statistic is the sum of the squared errors of the log odds ratio effects within the founder group in Fig. 2 and Supplementary Fig. 3 , and we permuted the founder membership of the isolates. We calculated P -values by Monte Carlo with 10,000 replications. Tests on the oocyst intensity used linear regression on the log counts, including main effects for flask (and hence isolate) and mosquito vector, and interaction effects between isolate and vector, with the overall test of interaction done by analysis of variance. Statistical analyses were done using R (Version 3.2.0). P -values <0.05 were deemed significant. Genotyping and population genetics Deep-sequencing data for 603 P. falciparum clinical isolates contributed by the authors were obtained by the MalariaGEN Plasmodium falciparum Community Project ( http://www.malariagen.net/projects/parasite/pf ). Full details of sample preparation, sequencing and genotyping are given elsewhere [12] . Briefly, DNA extracted from leukocyte-depleted venous blood was sequenced using the Illumina HiSeq platform and the resulting paired short reads were assembled and quality filtered to produce genotype calls for 681,587 high-quality variations. Genotype calls were supported by at least five sequencing reads, with at least two reads required to call individual alleles. These genotype calls were used to call K13 genotypes using a custom procedure [12] and to define Pfs47 haplotypes, which could be reconstructed without missingness in 516 samples. Parasites were classified into core and founder populations by a multi-stage clustering technique based on ancestry analysis, as previously described [12] . All nucleotide read sequences were deposited in the European Nucleotide Archive database ( http://www.ebi.ac.uk/ena ), where they are publicly accessible; a list of European Nucleotide Archive accession codes is given in Supplementary Data 1 . How to cite this article: St. Laurent, B. et al. Artemisinin-resistant Plasmodium falciparum clinical isolates can infect diverse mosquito vectors of Southeast Asia and Africa. Nat. Commun. 6:8614 doi: 10.1038/ncomms9614 (2015).